Inhibition of KRAS codon 12 mutants using a novel DNA-alkylating pyrrole–imidazole polyamide conjugate Despite extensive efforts to target mutated RAS proteins, anticancer agents capable of selectively killing tumour cells harbouring KRAS mutations have remained unavailable. Here we demonstrate the direct targeting of KRAS mutant DNA using a synthetic alkylating agent (pyrrole–imidazole polyamide indole- seco -CBI conjugate; KR12) that selectively recognizes oncogenic codon 12 KRAS mutations. KR12 alkylates adenine N3 at the target sequence, causing strand cleavage and growth suppression in human colon cancer cells with G12D or G12V mutations, thus inducing senescence and apoptosis. In xenograft models, KR12 infusions induce significant tumour growth suppression, with low host toxicity in KRAS-mutated but not wild-type tumours. This newly developed approach may be applicable to the targeting of other mutant driver oncogenes in human tumours. Recent advances in the next-generation sequencing of human tumours have uncovered hundreds of recurrent oncogenic driver mutations and have identified many novel, actionable therapeutic targets. Oncogenic driver genes, which are often mutated, are continuously expressed and thereby contribute to cancer cell survival, which is a target for clinical therapy. Targeting the RAS–MAPK pathway has led to the development of successful treatments of epidermal growth factor receptor-mutant cancers but has also revealed that unexpected degrees of oncogene addiction and signalling complexity exist [1] . A common outcome of treatment using inhibitors of genes that lie ‘downstream’ in the RAS pathway is the development of drug resistance [2] , and new approaches that target mutant RAS genes may provide a more direct route to inhibit these poor-prognosis tumours. RAS genes, particularly H-ras, N-ras and K-ras, were the first human oncogenes to be discovered in human tumours more than 30 years ago and are among the most commonly mutated and critical cancer driver genes. The legendary K-Ras protein has been on everyone’s ‘target’ list since its discovery. It has been estimated that ∼ 33,000 newly diagnosed colon cancer patients in the United States during the year 2013 had the KRAS (G12D) mutation, which is considered the most frequent mutation in metastatic colon cancer, or the (G12V) mutation [3] , [4] . Extensive efforts have therefore been made to develop one or more small chemical compounds that could directly target and inhibit constitutively active KRAS. Unfortunately, direct pharmacological targeting of activated KRAS has, to date, been unsuccessful for clinical use [5] . Recently, a G12C KRAS mutation has been successfully targeted in vitro by a small molecule that allosterically controls GTP affinity and effector interactions, representing a promising approach to therapy for this specific subset of KRAS mutant tumours [6] . In the face of the challenges in developing small-molecule drugs that directly target KRAS mutant proteins [7] , we have developed a novel approach that directly targets the mutant DNA. Hairpin pyrrole (Py)–imidazole (Im) (PI) polyamides can be designed to bind with high affinity to the minor groove of specific DNA sequences [8] : Py moieties preferentially bind T, A and C bases, but not G, whereas Im is a G-reader. These agents have shown efficacy in preclinical animal models of human diseases, including cancer, with minimal toxicity [9] , [10] , [11] . For example, PI polyamide conjugates with 1,2,9,9a-tetrahydrocyclopropa[1,2-c]benz[1,2-e]indol-4-one (CBI), which is converted to its cyclopropyl form via cyclization of a precursor containing a chloromethyl group to alkylate target DNA at the minor groove of N3 of adenine under neutral pH conditions, is a synthetic analogue of the alkylating moiety of duocarmycin A and can improve the limitations of targeting a coding sequence [12] , [13] , [14] . We therefore synthesized PI polyamide indole- seco -CBI conjugates to target common KRAS codon 12 mutations. KR12 targets KRAS codon 12 (G12D and G12V) mutants The compounds IPβIIPI-γ-PIβPP-indole- seco -CBI (KR12: Fig. 1a ) and IIPIβPI-γ-PIPβP-indole- seco -CBI (#6) [15] were designed and synthesized to recognize and alkylate adenine residues on the template strand of exon 2 of mutant KRAS, specifically at codon 12 (GTT and GAT) and codon 13 (GAC), respectively, according to the general recognition rule for PI polyamides [8] . 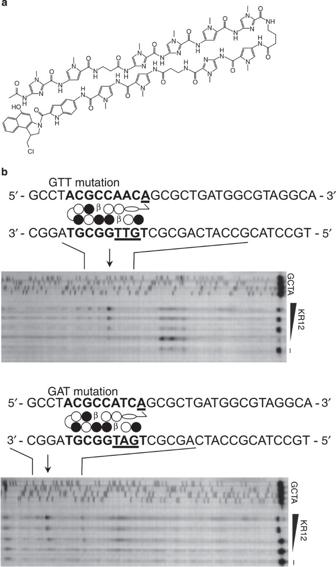Figure 1: Structure of KR12 and the sequence-specific cleavage of a DNA strand through KR12-dependent alkylation. (a) Chemical structure of the PI polyamideseco-CBI conjugate, termed KR12. (b) Schematic drawing of thermal-induced cleavage at the sites ofKRAScodon 12 mutations. The upper and lower panels represent the G12V;GTT and G12D;GAT mutations. Closed circles represent imidazole moieties and arrows indicate the positions of KR12-dependent alkylation and cleavage. An increased level of specific cleavage products was seen with increasing doses of KR12 (from bottom to top,b). The hairpin PI polyamide for KR12 but not for #6 preferentially bound to the mutant KRAS sequences, compared with wild-type, as shown by gel shift and surface plasmon resonance assays ( Supplementary Figs 1 and 2 , and Supplementary Table 1 ). Alkylation of theoretical recognition sequences, that is, 5′-WCGCCWWCA-3′ for KR12 and 5′-WCGWCWCCA-3′ for #6 (W indicates A or T), was confirmed using a thermally induced strand cleavage procedure [15] . Dose-dependent, alkylation-mediated selective DNA strand cleavage was detected at the G12D/G12V mutations in the presence of KR12 ( Fig. 1b ), and #6 showed specific cleavage of the sequence at the codon 13 mutation [15] . Strong, dose-dependent alkylation by KR12 was detected only at the mutated KRAS codon 12 target sites among ∼ 160 base pairs of KRAS EXON2 plus plasmid sequences, which did not have additional full-match recognition sites of KR12. Figure 1: Structure of KR12 and the sequence-specific cleavage of a DNA strand through KR12-dependent alkylation. ( a ) Chemical structure of the PI polyamide seco -CBI conjugate, termed KR12. ( b ) Schematic drawing of thermal-induced cleavage at the sites of KRAS codon 12 mutations. The upper and lower panels represent the G12V;GTT and G12D;GAT mutations. Closed circles represent imidazole moieties and arrows indicate the positions of KR12-dependent alkylation and cleavage. An increased level of specific cleavage products was seen with increasing doses of KR12 (from bottom to top, b ). Full size image The KR12-induced cell growth inhibition of a series of KRAS mutated or non-mutated human colon cancer cell lines, that is, HT29 (WT), Caco-2 (WT), SW1463 (12C/12C; GGT-TGT), SW480 (12V/12V; GGT-GTT), SW620 (12V/12V) and LS180 (12D; GGT-GAT/WT), were then analysed using the standard WST (water-soluble tetrazolium salts) assay. The viability of KRAS G12D or G12V mutant cells was significantly lower after treatment compared with wild-type cells or SW1463 cells carrying the G12C mutation, which is not recognized by KR12 ( Fig. 2a ; see also additional data on cell lines SNU-C2B (12D/12D) and DLD1 (13D/WT) in Supplementary Table. 2 ). A distinct pattern of cell viability was observed after KR12 treatment. Cell lines with KR12-recognized KRAS mutations (12D or 12V) were more sensitive than cell lines without those sequences, while there was no correlation between cell growth and p53 mutation status. 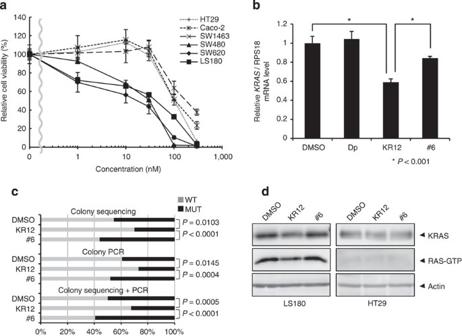Figure 2: KR12-mediated specific suppression of KRAS codon 12 mutants in human colon cancer cells. (a) WST assay. Human colon cancer cells expressing wild-type KRAS, including HT29 and Caco-2 or human colon cancer cells harbouringKRAScodon 12 mutations, including SW1643, SW480, SW620 and LS180, were incubated with the indicated concentrations of KR12. Forty-eight hours after treatment, the percent viable cells were examined by WST assay and depicted in a line graph. Error bars indicate the s.d. of the data from triplicate experiments. (b) Quantitative reverse transcription-PCR analysis. Relative KRAS expression 48 h after treatment with DMSO, KR12, #6 or Dp was plotted as a bar graph. Error bars indicate the s.d. of data from triplicate experiments. (c) Allele-specific downregulation ofKRAScodon 12 mutant: cDNA from the treated RNA was subcloned. Transfected antibiotic-resistant/colour-selected colonies were screened by colony PCR and direct colony-sequencing methods. The number of colonies for the wild-type or codon 12KRASmutant allele of each treated group was counted and reported inSupplementary Table 3. The percentages of wild-type and mutantKRASsequences are also shown in parentheses. (d) Immunoblot analysis. Immunoblots for anti-KRAS or anti-actin antibody (top and bottom panels, respectively) for LS180 (12D/WT) and HT29 (WT) cells 48 h after the treatment with either control DMSO solution, KR12 or #6. The GST-Raf-bound proteins from each treated group were pulled down and analysed by immunoblotting with anti-RAS antibody (middle panels). Figure 2: KR12-mediated specific suppression of KRAS codon 12 mutants in human colon cancer cells. ( a ) WST assay. Human colon cancer cells expressing wild-type KRAS, including HT29 and Caco-2 or human colon cancer cells harbouring KRAS codon 12 mutations, including SW1643, SW480, SW620 and LS180, were incubated with the indicated concentrations of KR12. Forty-eight hours after treatment, the percent viable cells were examined by WST assay and depicted in a line graph. Error bars indicate the s.d. of the data from triplicate experiments. ( b ) Quantitative reverse transcription-PCR analysis. Relative KRAS expression 48 h after treatment with DMSO, KR12, #6 or Dp was plotted as a bar graph. Error bars indicate the s.d. of data from triplicate experiments. ( c ) Allele-specific downregulation of KRAS codon 12 mutant: cDNA from the treated RNA was subcloned. Transfected antibiotic-resistant/colour-selected colonies were screened by colony PCR and direct colony-sequencing methods. 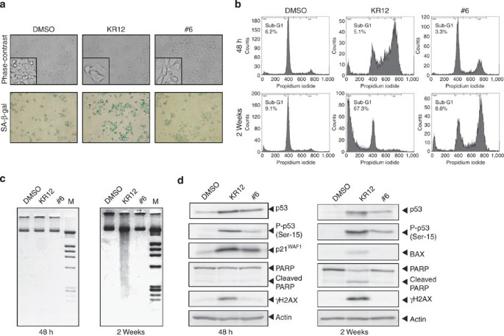Figure 3: KR12-dependent induction of cellular senescence and apoptosis. (a) SA-β-gal staining. LS180 cells were exposed to DMSO, KR12 or #6 (at a final concentration of 50 nM). Forty-eight hours after treatment, phase-contrast microphotographs were taken (top panels) and the cells were washed in PBS, fixed in 2% formaldehyde plus 0.05% glutaraldehyde and incubated with SA-β-gal staining solution containing X-gal for 24 h at 37 °C (bottom panels). (b) Cell cycle distribution analysis. Forty-eight hours (top) and two weeks (bottom) after treatment, cells were subjected to FACS analysis, and the DNA contents of each sample were analysed and depicted following the manufacturer's instructions. (c) DNA fragmentation. The attached and floating LS180 cells 48 h (left) and 2 weeks (right) after treatment were collected, and their genomic DNA was prepared and analysed by 1% agarose gel electrophoresis with λ/HindIII and φ-X174/HaeIII size markers. (d) Immunoblotting. Forty-eight hours (left) and 2 weeks (right) after the treatment, whole-cell lysates were prepared and subjected to immunoblotting with the indicated antibodies. Actin was used as a loading control. The number of colonies for the wild-type or codon 12 KRAS mutant allele of each treated group was counted and reported in Supplementary Table 3 . The percentages of wild-type and mutant KRAS sequences are also shown in parentheses. ( d ) Immunoblot analysis. Immunoblots for anti-KRAS or anti-actin antibody (top and bottom panels, respectively) for LS180 (12D/WT) and HT29 (WT) cells 48 h after the treatment with either control DMSO solution, KR12 or #6. The GST-Raf-bound proteins from each treated group were pulled down and analysed by immunoblotting with anti-RAS antibody (middle panels). Full size image Mutant KRAS suppression induced by KR12 To analyse the specific alkylation and subsequent downregulation of the KRAS mutant allele after KR12 treatment, human colon cancer-derived, heterozygously mutated LS180 (12V/WT) cells were used to evaluate allele-specific suppression after dimethyl sulfoxide (DMSO), KR12, #6 or KR12 lacking seco -CBI (Dp) treatment. Endogenous DNA alkylation at the KRAS codon 12 mutation in LS180 cells after KR12 but not after #6 or DMSO treatment was repeatedly confirmed using ligation-mediated PCR ( Supplementary Fig. 3 ). Unlike DMSO-, #6- or Dp-treated cells, KR12-treated cells showed significant downregulation of total KRAS and mutated KRAS allele expression by quantitative reverse transcription-PCR and colony PCR/sequencing assays, respectively ( Fig. 2b,c and Supplementary Table 3 ). Immunoblot analysis also revealed that KR12, but not #6, induced a significant reduction in KRAS protein levels and in its GST-Raf-bound, active GTP-bound form, whereas KR12 had an undetectable effect on KRAS levels or activity in HT29 cells harbouring wild-type KRAS ( Fig. 2d ). In contrast to KR12, Dp had an undetectable effect on KRAS codon 12 mutant expression, indicating that the targeted hairpin PI polyamide lacking the CBI alkylating moiety was not sufficient to reduce the expression of the targeted mutant gene ( Fig. 2b ). Induction of 12V mutation sequence-specific alkylation after KR12 treatment could induce specific reductions in mutated KRAS RNA and in activated KRAS protein levels in heterozygous LS180 cells. We also observed slight reduction of KRAS downstream proteins of phospho-AKT and phospho-ERK expression after KR12 treatment ( Supplementary Fig. 4d ). Senescence and DNA damage induced by KR12 in LS180 cells We next investigated the biological effects of KR12 on KRAS mutant colon carcinoma cells. After 48 h of 50 nM KR12 treatment, a flat cell morphology was displayed in LS180 cells, and SA-β-gal activity was strongly increased compared with DMSO- or #6-treated cells, suggesting that KR12 induced cellular senescence ( Fig. 3a ). Cellular senescence is a stress response that stably blocks proliferation induced by activation of the RAS pathway, but is dependent on the cellular context [16] . Cell cycle arrest is a critical process in cellular senescence that is induced by the CDK inhibitor p21 WAF1/CIP1 (ref. 17 ), and 48-h KR12 exposure significantly increased the proportion of G2/M-phase cells ( Fig. 3b ). In contrast, DMSO and #6 had less of an effect on cell cycle distribution, and none of the three treatments increased the number of sub-G1-phase cells or the level of apoptotic genomic DNA fragmentation ( Fig. 3c ). KR12 markedly induced phosphorylation of p53 at Ser-15, p21 WAF1/CIP1 and phosphorylated histone variant H2AX (γH2AX), whereas KR12-mediated cleavage of PARP at the 48-h time point was not observed ( Fig. 3d ). Phospho-p53 (Ser-15) and γH2AX inductions in KR12-treated cells were also visually confirmed by indirect immunofluorescence staining ( Supplementary Fig. 4b ). We conclude that KR12 promotes p53-dependent cellular senescence, which is an important tumour suppressor mechanism [16] , as well as DNA double-strand breaks, but not apoptosis, after short-term treatment. Figure 3: KR12-dependent induction of cellular senescence and apoptosis. ( a ) SA-β-gal staining. LS180 cells were exposed to DMSO, KR12 or #6 (at a final concentration of 50 nM). Forty-eight hours after treatment, phase-contrast microphotographs were taken (top panels) and the cells were washed in PBS, fixed in 2% formaldehyde plus 0.05% glutaraldehyde and incubated with SA-β-gal staining solution containing X-gal for 24 h at 37 °C (bottom panels). ( b ) Cell cycle distribution analysis. Forty-eight hours (top) and two weeks (bottom) after treatment, cells were subjected to FACS analysis, and the DNA contents of each sample were analysed and depicted following the manufacturer's instructions. ( c ) DNA fragmentation. The attached and floating LS180 cells 48 h (left) and 2 weeks (right) after treatment were collected, and their genomic DNA was prepared and analysed by 1% agarose gel electrophoresis with λ/ Hind III and φ-X174/ Hae III size markers. ( d ) Immunoblotting. Forty-eight hours (left) and 2 weeks (right) after the treatment, whole-cell lysates were prepared and subjected to immunoblotting with the indicated antibodies. Actin was used as a loading control. Full size image p53-dependent apoptosis is induced by KR12 in LS180 cells Strong induction of apoptosis was, however, observed in LS180 cells after 14 days of continuous 50 nM KR12 treatment, as evidenced by the significant increase in sub-G1-phase cells shown by fluorescence-activated cell sorting (FACS) analysis ( Fig. 3b and Supplementary Fig. 4a ) and typical DNA fragmentation ( Fig. 3c ), while #6 induced G2/M arrest. LS180 cells, which carry hemizygous wild-type p53 (ref. 18 ), showed marked induction of p53 in association with cleaved PARP accumulation and γH2AX, while treatment with #6 resulted in faint p53 activation without PARP cleavage ( Fig. 3d ), implying that apoptosis induction by long-term KR12 treatment might be p53 dependent. The induction of p53 phosphorylation at Ser-15 and of γH2AX was also visually confirmed by indirect immunofluorescence staining ( Supplementary Fig. 4c ). On the basis of these data, we propose that treatment of LS180 cells with KR12, but not with #6, introduces DNA breaks at the KRAS locus and induces γH2AX foci and senescence and that after extended exposure to the drug, apoptosis occurs. KRAS knockdown enhances DNA alkylator-induced cell death To confirm a possible synergy of DNA alkylator and KRAS suppression in LS180 cells, we assessed LS180 growth inhibition after treatments with short interfering RNA (siRNA) targeting KRAS, control siRNA, #6 (KRAS non-targeting PI polyamide-indole- seco -CBI) and combinations of siRNAs and #6. Although single treatments with either KRAS siRNA or #6 with control siRNA resulted in reduced LS180 cell viability, 1 nM of KRAS siRNA induced a partial reduction of cell growth. When treated together with a low dose (0.3 nM) of #6, 1 nM of KRAS siRNA resulted in significantly higher cell growth reduction than samples treated with 1 nM of control siRNA ( Supplementary Fig. 5a,b ), implying that even partial reduction of KRAS and its downstream signals may sufficiently increase the sensitivity of alkylating agents in LS180 cells. KR12 also caused the partial downregulation of the active KRAS mutant and of DNA alkylation induction; therefore, KR12 increases its own ability to induce DNA damage, which is followed by cell death, in a similar manner. Preferential in vivo tumour growth reduction by KR12 The potential efficacy of KR12 in vivo was tested by weekly intravenous injection of DMSO or KR12 (320 μg kg −1 ) for 5 weeks into nude mice inoculated with HT29 (KRAS WT), LS180 (heterozygous 12D/WT) or SW480 (homozygous 12V) cells. 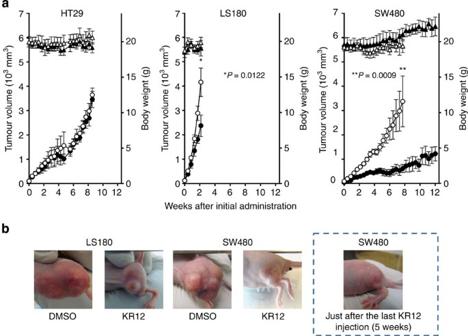Figure 4: KR12 suppresses tumour growthin vivo. (a) The indicated human colon cancer cells, that is, HT29 (WT), LS180 (12D/WT) and SW480 (12V/12V), were injected subcutaneously into BALB/c nude mice. When the tumour volume reached 100 mm3, DMSO or KR12 (320 μg kg−1body weight) was intravenously injected through the tail vein every 7 days. At the indicated times after administration, the tumour volume was calculated as 1/6 π × the longest diameter × width × height. The mean tumour volume, with s.e. (open circles for DMSO and closed circles for KR12 treatment), and mean body weight, with s.e. (open triangles for DMSO and closed triangles for KR12 treatment), of the KR12-treated group and control group are plotted in a line graph with error bars (s.e.). The numbers of animals used were 6 for HT29 (DMSO and KR12) and LS180 (KR12), 5 for LS180 (DMSO) and SW480 (KR12), and 8 for SW480 (DMSO). (b) Images of the euthanized mice of each group are shown. An image of an SW480 xenograft 5 weeks after KR12 treatment, which was the final treatment, is also shown. Treatment was started when the tumour size reached 100 mm 3 ( Supplementary Table 4 and Supplementary Fig. 6a ). KR12 injection had an undetectable effect on the growth of HT29 tumours, whereas a significant reduction of tumour growth, with minimum toxicity, was demonstrated for the SW480 ( P =0.0009) and LS180 ( P =0.0122) tumours on significantly reducing KRAS expression in those tumours ( P =0.0388; Fig. 4 and Supplementary Figs 6b and 7b ). Even after cessation of treatment at 5 weeks, KR12-treated SW480 tumours consistently showed slower growth than the DMSO-treated controls ( Supplementary Fig. 7a ). Furthermore, the KR12-treated SW480 tumours exhibited movable, hard fibrotic nodules. We also examined the same experiment using an alkylating agent of CBI itself and #6, which should not have performed specific alkylation at the KRAS 12D mutation. Although CBI showed a strong antitumour effect, this tumour growth reduction was slightly weaker than that from KR12 treatment, and #6 did not show any significant antitumour effects in the SW480 xenografted nude mouse model. It was also intriguing that mice treated with KR12, #6 or DMSO remained healthy during the experiment, while CBI-treated mice exhibited weight loss and slight illness ( Supplementary Fig. 7a ). Figure 4: KR12 suppresses tumour growth in vivo . ( a ) The indicated human colon cancer cells, that is, HT29 (WT), LS180 (12D/WT) and SW480 (12V/12V), were injected subcutaneously into BALB/c nude mice. When the tumour volume reached 100 mm 3 , DMSO or KR12 (320 μg kg −1 body weight) was intravenously injected through the tail vein every 7 days. At the indicated times after administration, the tumour volume was calculated as 1/6 π × the longest diameter × width × height. The mean tumour volume, with s.e. (open circles for DMSO and closed circles for KR12 treatment), and mean body weight, with s.e. (open triangles for DMSO and closed triangles for KR12 treatment), of the KR12-treated group and control group are plotted in a line graph with error bars (s.e.). The numbers of animals used were 6 for HT29 (DMSO and KR12) and LS180 (KR12), 5 for LS180 (DMSO) and SW480 (KR12), and 8 for SW480 (DMSO). ( b ) Images of the euthanized mice of each group are shown. An image of an SW480 xenograft 5 weeks after KR12 treatment, which was the final treatment, is also shown. Full size image Although other drugs have been developed against the RAS signalling pathway, they are mainly effective against cancers with wild-type KRAS and are often ineffective in the treatment of KRAS-mutated colorectal cancers [19] . The PI polyamide-based alkylation strategy specifically downregulated constitutively active KRAS and efficiently suppressed the in vitro growth of several KRAS mutant cancer cell lines through the induction of DNA damage and cellular senescence followed by apoptosis. The in vivo growth of KRAS G12V/G12D mutant tumour xenografts was also efficiently suppressed by weekly injections of KR12 into mice bearing tumours induced by the inoculation of LS180 or SW480 cells. Therefore, KR12 is a promising anticancer drug candidate for unmet KRAS codon 12 mutant cancers. We propose that PI polyamide-mediated-specific silencing of mutant oncogenic driver genes may therefore facilitate the development of a pipeline of next-generation, molecular-targeted therapeutic strategies that could be applied in combination with mutant driver gene identification by sequencing the exomes of human cancers as a route to ‘Precision Medicine’ that is targeted at the individual patient. Hairpin N -methylpyrrole(Py)- N -methylimidazole(Im) polyamide indole- seco -CBI conjugates [12] , [13] can be designed for specific 9-base-pair recognition of the genome following Dervan’s recognition rule, as seen in natural minor groove binders, which undergo hydrogen bonding to DNA [8] . Under neutral pH, the open-ringed seco -CBI moiety is converted to CBI, which then alkylates the N3 of adenine in the DNA minor groove. When conjugated to PI polyamide indole, the conjugates increase sequence recognition specificity compared with conventional alkylating agents, which mainly recognize the N6 of guanine in the DNA major groove without recognizing the genomic DNA sequence [12] , [13] , [14] , [20] . Although indole, γ-aminobutyric acid (γ-turn) and beta-alanine linker may require optimization to improve their specificity and sensitivity for sequence-specific alkylation, the recognition of specific 9-bp sites in the genome by KR12 allows for multiple recognition sites ( ∼ 9,121 sites in the human genome (GRCh38/hg38)), where the mutated KRAS site should be included for preferential alkylation. KR12 treatment resulted in a significant reduction of activated KRAS and a significant induction in DNA damage followed by cell death in KRAS-mutated colon cancer cells. We observed dose-dependent alkylation at the mutated sequences by CBI conjugates, with approximately a 10-fold difference in the dissociation constants of the mutant and wild-type allele sequences, a reduction of mutant KRAS expression in heterozygous LS180 cells, endogenous alkylation of the KRAS mutant genome and in vitro and in vivo growth reduction of tumour cells with the KRAS mutations. All together, these results suggest that the DNA sequence-specific alkylating activity of hairpin polyamide indole- seco -CBI recognizes the match sequence instead of the mismatch site. The number of naked PI polyamides showing biological efficacy as single agents remains limited. Thus, one way to enhance the therapeutic potential of PI polyamides might be to conjugate them to small-molecule drugs, such as alkylating agents [21] , [22] . In many clinical trials, chemotherapy and targeted therapy combinations result in better outcomes for patients and prolong overall survival. As KR12 is an alkylating agent targeting a restricted number of genomic regions, including the KRAS driver oncogene mutation, it appears suited for combination therapy between molecular-targeted therapy and conventional chemotherapy. Because of the sequence-specific DNA recognition of KR12, the number of genomic regions that are alkylated by KR12 should also be dramatically reduced in comparison with conventional chemotherapy; therefore, the adverse effect of toxicity to normal cells may be remarkably reduced, as demonstrated in animal experiments ( Supplementary Fig. 7a ). Although potential off-target effects of KR12 should exist among the 9,121 estimated target sites in the reference human genome (GRCh38/hg38), this possibility may not be a major concern for cancer patients with poor prognosis and experience with conventional chemotherapy. Although many issues still remain to be addressed for the clinical development of PI polyamide-indole- seco -CBI, as usually seen in cases of drug development, targeting oncogenic driver genes for alkylation may promise a fruitful feature of cancer therapy for untreatable cancer patients with unfavourable prognoses. Extensive genomic sequencing of tumour and normal tissues may provide critical biomarkers to aid in finding appropriate cancer cases that should be treated by KR12 or another specific genome-targeting alkylator. Tumour selectivity is another important issue for anticancer treatment. In contrast to traditional cytotoxic chemotherapies, which crudely target growth processes shared by normal and cancerous tissues, agents such as imatinib mesylate (Gleevec) for BCR–ABL translocation that target genetic alterations underlying cancer often have mild toxicity because of their greater specificity for cancer cells [23] . In addition to specificity to the cancer genome, PI polyamide has been reported to accumulate specifically in xenografted tumour tissue in some cases [24] . These unique properties of PI polyamide conjugates provide a very efficient capacity for drug delivery, and its alkylating conjugate, which targets oncogenic somatic mutations, could reveal a superb selective advantage by specifically targeting cancer cells with the mutation. This possibility may also support the observed very specific and effective in vivo anticancer activity of KR12. In conclusion, a synthetic PI polyamide alkylator conjugate of KR12 has been designed to target KRAS mutations and induce mutant KRAS suppression followed by tumour cell death in vitro and in vivo in an oncogenic mutation-specific manner. Thus, KR12 is a possible candidate drug for colorectal patients with either the G12D or G12V mutation. Compounds The compounds ImPyβImImPyIm-γ-PyImβPyPy-indoleCBI (KR12), shown in Fig. 1a , and ImPyβImImPyIm-γ-PyImβPyPy-indoleCBI (#6) [15] were designed and synthesized as described previously [20] . In brief, PI polyamides were synthesized in a stepwise reaction using a previously described Fmoc solid-phase protocol [12] and a peptide synthesizer (PSSM-8, Shimadzu Industry) with a computer-assisted operation system on a 10-μmol scale (9.8 mg of Fmoc-β-alanine Wang resin). After synthesis, 1 ml of 50% 1N LiOH/NMP was mixed with the resin and the mixture was heated at 55 °C for 1 h to detach the PI polyamides from the resin. The PI polyamides were then purified by high-performance liquid chromatography (HPLC) LC-20 (Shimadzu Industry) using a 10 × 150 mm Phenomenex Gemini-NX3u 5-ODS-H reverse-phase column in 0.1% acetic acid in water, with acetonitrile as the eluent, a flow rate of 10 ml min −1 , a linear gradient from 30 to 75% acetonitrile over 30 min and detection at 310 nm. Collected KR12-COOH fractions were analysed by LC-MS. DIEA (0.5 μl, 2.86 μmol) and PyBOP (1.0 mg, 1.95 μmol) were added to a solution of Py–Im polyamide carboxylic acid KR12-COOH (1.0 mg, 0.66 μmol) in NMP (100 μl) and the reaction mixture was stirred for 1 h at room temperature. After conversion from KR12-COOH to the activated 1-hydroxybenzotriazole ester was verified by analytical HPLC (0.1% TFA/CH3CN 30–75% linear gradient, 0–30 min), NH 2 -indole- seco -CBI (0.6 mg, 1.58 μmol) was added to the reaction vessel and the reaction mixture was stirred for 4 days at room temperature. The reaction mixture was subjected to HPLC purification (0.1% TFA/CH 3 CN 30–75% linear gradient, 0–30 min), and the peak fraction containing the product was collected. After lyophilization, KR12 was produced as a white powder. High-resolution gel electrophoresis 5′-Texas Red-labelled DNA fragments containing the indicated KRAS codon 12 mutations were incubated with the indicated concentrations of KR12 for 10 h at room temperature, followed by the addition of calf thymus DNA. The reaction mixtures were then incubated at 90 °C for 5 min to cleave DNA strands at their specific alkylated sites. DNA fragments were then recovered by vacuum centrifugation, dissolved in loading dye, denatured at 95 °C for 20 min and subjected to electrophoresis on a 6% denaturing polyacrylamide gel. Cell culture Human colon carcinoma-derived HT29 (WT), Caco-2 (WT), SW1463 (12C/12C), SW480 (12V/12V) and SW620 (12V/12V) cells were maintained in Dulbecco’s modified Eagle’s medium supplemented with heat-inactivated 10% fetal bovine serum, 100 U ml −1 of penicillin and 100 μg ml −1 of streptomycin. Human colon carcinoma-derived LS180 (12D/WT) cells were grown in Eagle’s minimum essential medium containing heat-inactivated 10% fetal bovine serum, 100 U ml −1 of penicillin and 100 μg of streptomycin. All cell lines were cultured in a 37 °C humidified atmosphere containing 95% air and 5% CO 2 . Cell proliferation analysis Cells were seeded at a final density of 3 × 10 3 or 5 × 10 3 cells per 96-well plate and allowed to attach overnight. The cells were then treated with 0.125% DMSO, 50 nM KR12 or #6. Forty-eight hours after treatment, 10 μl of WST-8 reagent (Dojindo) was added to each culture and the reaction mixtures were incubated at 37 °C for another 2 h. The absorbance readings for each well were performed at 450 nm using a microplate reader (MTP-310; Corona). Real-time reverse-transcriptase PCR Total RNA was prepared using the RNAeasy plus mini kit according to the manufacturer’s instructions (Qiagen), and 0.5 μg of the RNA was converted to cDNA using the SuperScript VILO cDNA Synthesis System (Invitrogen) according to the manufacturer’s protocols. The q-PCR Master Mix and specific primer sets were used for SYBR Green-based quantitative PCR (q-PCR; Applied Biosystems). Three independent measurements were taken and the amounts were estimated by extrapolation from a standard curve. Expression values were normalized against the expression of RPS18 and used as an endogenous control. The primer sets used in this study were as follows: KRAS, 5′-GGAGAGAGGCCTGCTGAA-3′ (sense) and 5′-TGACCTGCTGTGTCGAGAAT-3′ (antisense); and RPS18 , 5′-GAGGATGAGGTGGAACGTGT-3′ (sense) and 5′-TCTTCAGTCGCTCCAGGTCT-3′ (antisense). RAS GTP assay Cells were washed twice in ice-cold PBS and lysed in Mg 2+ lysis buffer (MLB; Millipore) and protein concentrations were measured using the Bio-Rad Protein Assay System (Bio-Rad). Equal amounts of cell lysates (500 μg of protein) were mixed with 10 μl of GST-Raf-conjugated agarose beads (Millipore) and incubated for 45 min at 4 °C. After incubation, the agarose beads were extensively washed in lysis buffer and boiled in 40 μl of 2 × SDS-sample buffer for 5 min, and the supernatants were analysed by immunoblotting with anti-KRAS antibody (Abcam, ab55391). Immunoblot analysis Equal amounts of cell lysates prepared from LS180 cells exposed to DMSO, KR12 or #6 were separated by 10% SDS–polyacrylamide gel electrophoresis and electrotransferred onto polyvinylidene difluoride membranes (Immobilon-P; Millipore). The membranes were blocked with TBS-T (Tris-buffered saline plus 0.05% Tween 20) containing 5% non-fat dry milk. After blocking, the membranes were incubated with anti-KRAS (ab55391, Abcam, 1:1,000), anti-p21 WAF1 (sc-756, Santa Cruz Biotechnology, 1:1,000), anti-p53 (sc-126, Santa Cruz Biotechnology, 1:4,000), anti-phospho-p53 at Ser-15 (9284, Cell Signaling Technology, 1:1,000), anti-PARP (9542, Cell Signaling Technology, 1:1,000), anti-γH2AX (613402, BioLegend, 1:2,000), anti-Actin antibody (A5060, Sigma, 1:2,000) or anti-BAX (2774, Cell Signaling Technology, 1:1,000) followed by incubation with the appropriate HRP (horseradish peroxidase)-conjugated secondary antibody (rabbit:7074, mouse:7076, Cell Signaling Technology). Following extensive washing in TBS-T, antibodies bound to the indicated proteins were visualized using enhanced chemiluminescence reagents (ECL; GE Life Sciences). Indirect immunofluorescence assay LS180 cells treated with DMSO, KR12 or #6 were rinsed twice in ice-cold PBS and then fixed in 3.7% formaldehyde at room temperature for 30 min. After washing in PBS, the cells were permeabilized with 0.1% Triton-X-100 in PBS at room temperature for 5 min and then blocked with 3% bovine serum albumin in PBS at room temperature for 1 h. After washing in PBS, the cells were incubated with anti-phospho-p53 at Ser-15 or with anti-γH2AX at room temperature for 1 h, followed by incubation with FITC-conjugated anti-rabbit IgG or rhodamine-conjugated anti-mouse IgG (Invitrogen), respectively, at room temperature for 1 h. The glass coverslips were washed in PBS and mounted with VectaShield containing DAPI (Vector Laboratories). Fluorescent images were captured using a confocal microscope (Leica). Flow cytometry Cell cycle distribution was examined by flow cytometric analysis with a FACScan flow cytometer (BD Biosciences) following the manufacturer’s instructions. In brief, the attached and floating cells were collected and fixed in ice-cold 70% ethanol. The cells were then stained with a solution containing 50 μg ml −1 of propidium iodide and 100 μg ml −1 of RNase A in PBS at 37 °C for 30 min to determine the total DNA content. The cell cycle distribution was then analysed using a FACScan flow cytometer. Animal tumour models The animal protocol was approved by Chiba Cancer Center Animal Ethics Committee. HT29 (WT), LS180 (12D/WT) or SW480 (12V/12V) cells were implanted subcutaneously into the dorsal flanks of 6-week-old female athymic mice ( Supplementary Fig. 6a ). When the tumour volume reached 100 mm 3 , administration of a non-toxic dose of DMSO or KR12 (320 μg kg −1 body weight) was performed and five subsequent weekly injections with DMSO or KR12 were administered through their tail veins. Tumour-bearing mice were euthanized at the indicated times over 12 weeks after the first administration or when the tumours exceeded 2 cm in diameter. Statistical evaluation Statistical analyses of the experimental data were performed using Student’s t -test. The statistical significance of tumour growth between the treated and control groups was assessed using the statmod software package for R ( http://www.w.r-project.org ) [25] . The significance level is set at a P value of <0.05. How to cite this article: Hiraoka, K. et al. Inhibition of KRAS codon 12 mutants using a novel DNA-alkylating pyrrole–imidazole polyamide conjugate. Nat. Commun. 6:6706 doi: 10.1038/ncomms7706 (2015).